The palindromic DNA-bound USP/EcR nuclear receptor adopts an asymmetric organization with allosteric domain positioning Nuclear receptors (NRs) regulate gene expression through DNA- and ligand-binding and thus represent crucial therapeutic targets. The ultraspiracle protein/ecdysone receptor (USP/EcR) complex binds to half-sites with a one base pair spaced inverted repeat (IR1), a palindromic DNA response element (RE) reminiscent of IRs observed for vertebrate steroid hormone receptors. Here we present the cryo electron microscopy structure of the USP/EcR complex bound to an IR1 RE which provides the first description of a full IR-bound NR complex. The structure reveals that even though the DNA is almost symmetric, the complex adopts a highly asymmetric architecture in which the ligand-binding domains (LBDs) are positioned 5′ off-centred. Additional interactions of the USP LBD with the 5′-flanking sequence trigger transcription activity as monitored by transfection assays. The comparison with DR-bound NR complexes suggests that DNA is the major allosteric driver in inversely positioning the LBDs, which serve as the main binding-site for transcriptional regulators. The ecdysone receptor (EcR) is a nuclear receptor (NR) involved in ecdysteroid-dependent insect development and reproduction. The ecdysone response elements (EcREs) found in the promoter region of target genes generally consist of imperfect inverted repeats of two degenerated AG(G/T)TCA half-sites spaced by a single base pair (IR1) [1] , [2] , [3] , [4] , [5] , [6] . The usage of palindromic sequences distinguishes the invertebrate USP (ultraspiracle protein)/EcR receptor from its vertebrate RXR- (retinoid X receptor) heterodimeric counterparts, whose DNA-binding sites are composed primarily of inherently asymmetric, polar half-sites arranged as direct repeats (DRs) [7] . Among vertebrate NRs, steroid hormone receptors (SHRs) also bind to palindromic sequences, which contain partially degenerated AGGTCA and AG(G/A)ACA half-sites spaced by 3 bps (IR3); SHRs such as oestrogen receptors (ER) and androgen receptors represent major pharmaceutical targets for which no structural information is available as full complexes. Because of the similarity of IRs reminiscent of those observed for vertebrate SHRs, as opposed to DR REs, USP/EcR provides an attractive model for the understanding of the topology of NRs bound to IR REs. Recent work has provided first structural insights into full NRs bound to DR REs (the first named NR–DNA binding domain, DBD, defines the 5′ position within the RE on the leading DNA strand) such as PPAR/RXR-DR1 [8] , [9] , HNF4-1α-DR1 [10] , RXR/RAR-DR2 & RXR/RAR-DR5 [9] and RXR/VDR-DR3 (VDR, vitamin D receptor) [11] ; other NRs such as RXR/TR and RXR/LXR bind to DR4 REs. However, there are no structures available of NRs bound to IR REs, a lack that we address here by the description of the first full IR-bound NR complex. The structure shows that the overall organization is asymmetric, despite the symmetric nature of the bound DNA. Structure of the USP/EcR/DNA complex The USP/EcR/DNA complexes have been reconstituted from purified Heliothis virescens USP and EcR ΔAB receptors (lacking only the highly variable and unstructured AB domains). To assign the polarity of the protein complex on the DNA, we determined the structures of three DNA complexes of USP/EcR, one with the core IR RE, and two with 5′- and 3′-extended DNAs, respectively ( Fig. 1 ). The core DNA complex was formed with a 19 bp DNA comprising the imperfect IR1 EcRE from the well-characterized heat-shock protein 27 ( hsp27 ) gene promoter [5] (see Methods and Supplementary Fig. 1 ). The structure of this complex was determined by single particle cryo-EM and 3D reconstruction to about 11 Å resolution ( Figs 1 and 2 and Supplementary Figs 2 and 3 ). It reveals a rather extended, non-compact structure ( Fig. 2a ) remarkably similar to the one found by small-angle X-ray diffraction (SAXS; Fig. 2g–i and Supplementary Fig. 4 ); in contrast, previously published crystal structures of NR complexes [8] , [10] , although differing significantly from each other, are altogether more compact, with PPAR/RXR showing the largest differences due to its closed conformation ( Fig. 2j ) as opposed to its conformation in solution as pointed out using SAXS [9] . The recent structure of the RXR/LXR/DR4 complex [12] is yet different from PPAR/RXR and more similar to RXR/VDR/DR3 (published while this publication was under review). We interpreted the cryo-EM map of the USP/EcR/DNA complex by fitting the individually known crystal structures of the USP/EcR ligand-binding domain (LBD) heterodimer and DBD/DNA complexes ( Supplementary Fig. 5 [13] , [14] ). The fitting was rather straightforward ( Fig. 2a ) because of the good quality of the cryo-EM map and because no conformational adjustments of the LBD and DBD structures were needed, suggesting that the individual domain structures are maintained in the full assembly. 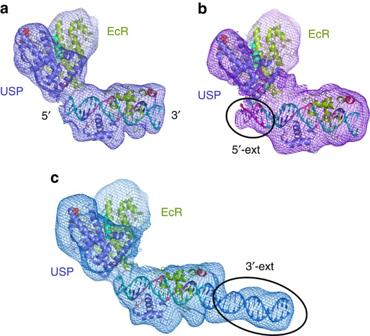Figure 1: Cryo-EM structures of the three USP/EcR DNA complexes. Cryo-EM maps and fitted models of the USP/EcR complexes with hsp27 DNA (a), 5′-hsp27 (b) and hsp27-3′ (c) DNAs extended by 5 and 18 base pairs, respectively (highlighted by oval marks) to annotate the 5′/3′ DNA polarity of the complex (with respect to the leading strand) and address interactions on the 5′ side of the core RE. Figure 1: Cryo-EM structures of the three USP/EcR DNA complexes. Cryo-EM maps and fitted models of the USP/EcR complexes with hsp27 DNA ( a ), 5′-hsp27 ( b ) and hsp27-3′ ( c ) DNAs extended by 5 and 18 base pairs, respectively (highlighted by oval marks) to annotate the 5′/3′ DNA polarity of the complex (with respect to the leading strand) and address interactions on the 5′ side of the core RE. 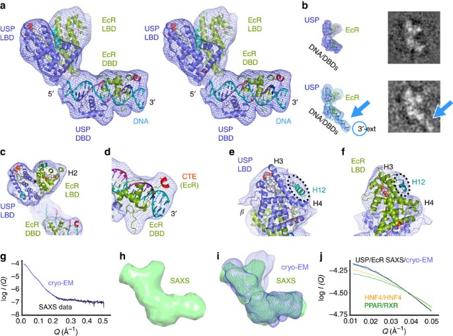Figure 2: Structure of the USP/EcR/IR1 DNA nuclear receptor complex. (a) Stereo representation of the USP/EcR/hsp27complex. The cryo-EM map is shown in magenta, with the fit of the individually available crystal structures of the DBD/DNA and LBD heterodimers. The DBDs of USP (blue) and EcR (green) are bound below and in front (side-on) of the DNA (drawn in-plane of the image), with the 5′ DNA end of the leading DNA strand on the left. (b) Class averages of the USP/EcR/hsp27and USP/EcR/hsp27-3′ complexes with the corresponding maps, revealing a density corresponding to the 18 bp DNA extension on the 3′ side. (c–f) Detailed views of the USP/EcR/hsp27complex regarding the USP and EcR LBDs, the EcR CTE helix and the antagonist and agonist positions of helix H12 in the USP and EcR LBDs, respectively. (g) Scattering curve (blue) computed from the USP/EcR/hsp27cryo-EM structure, which is in excellent agreement with the experimental X-ray scattering pattern (black) for the whole range of momentum transfer 0.01<Q<0.5 Å−1(whereQ=4π sin(θ)/λ, where 2θis the scattering angle andλis the wavelength) with aχ2=1.54, suggesting the same conformation in solution as analysed by SAXS or cryo-EM. (h,i)Ab initioenvelope of the USP/EcR/hsp27complex (light green) calculated withDAMMIF, and comparison with the cryo-EM map. (j) Comparison of the USP/EcR/hsp27experimental X-ray scattering pattern (black) and calculated scattering curve (blue) of the cryo-EM structure with the scattering curves calculated from the PPAR/RXR-DR18and HNF4-1α-DR1 crystal structures10, which differ significantly at small scattering angles, where PPAR/RXR-DR1 is much less compact in solution than in the crystal9, whereas the RXR/LXR/DR4 complex12is different from PPAR/RXR and more similar to RXR/VDR/DR3 (ref.11). Full size image Figure 2: Structure of the USP/EcR/IR1 DNA nuclear receptor complex. ( a ) Stereo representation of the USP/EcR/ hsp27 complex. The cryo-EM map is shown in magenta, with the fit of the individually available crystal structures of the DBD/DNA and LBD heterodimers. The DBDs of USP (blue) and EcR (green) are bound below and in front (side-on) of the DNA (drawn in-plane of the image), with the 5′ DNA end of the leading DNA strand on the left. ( b ) Class averages of the USP/EcR/ hsp27 and USP/EcR/ hsp27 -3′ complexes with the corresponding maps, revealing a density corresponding to the 18 bp DNA extension on the 3′ side. ( c – f ) Detailed views of the USP/EcR/ hsp27 complex regarding the USP and EcR LBDs, the EcR CTE helix and the antagonist and agonist positions of helix H12 in the USP and EcR LBDs, respectively. ( g ) Scattering curve (blue) computed from the USP/EcR/ hsp27 cryo-EM structure, which is in excellent agreement with the experimental X-ray scattering pattern (black) for the whole range of momentum transfer 0.01< Q <0.5 Å −1 (where Q =4π sin( θ )/ λ , where 2 θ is the scattering angle and λ is the wavelength) with a χ 2 =1.54, suggesting the same conformation in solution as analysed by SAXS or cryo-EM. ( h,i ) Ab initio envelope of the USP/EcR/ hsp27 complex (light green) calculated with DAMMIF , and comparison with the cryo-EM map. ( j ) Comparison of the USP/EcR/ hsp27 experimental X-ray scattering pattern (black) and calculated scattering curve (blue) of the cryo-EM structure with the scattering curves calculated from the PPAR/RXR-DR1 [8] and HNF4-1α-DR1 crystal structures [10] , which differ significantly at small scattering angles, where PPAR/RXR-DR1 is much less compact in solution than in the crystal [9] , whereas the RXR/LXR/DR4 complex [12] is different from PPAR/RXR and more similar to RXR/VDR/DR3 (ref. 11 ). Full size image The molecular model derived from the cryo-EM data provides important insights into the full USP/EcR complex ( Fig. 2 ). With respect to an orientation perpendicular to the DNA, the LBDs are slightly tilted (~20°) towards the 5′ direction and rotated by ~30° around the pseudo-two-fold symmetry axis that goes through the LBD interface of USP and EcR ( Fig. 2c ). This results in an asymmetric arrangement where the USP LBD is closer to the DNA than the EcR LBD ( Fig. 2a ). The LBDs have their N-terminal end oriented towards the DNA, whereas the ligand-binding pockets [13] , [15] are oriented away from the DNA ( Fig. 2a ). Although the LBDs of USP and EcR are pseudo-symmetric (see view on the pseudo-two-fold symmetry axis in Fig. 2c ) they can be distinguished unambiguously in the cryo-EM map thanks to specific structural differences, for example the EcR-specific helix H2 ( Fig. 2c ) and the ß-sheet region of USP that protrude from the LBD core (not fully visible in the crystal structure; Fig. 2e ). The structure shows that helix H12 of EcR is in the agonist position (due to presence of the ecdysteroid ligand; Fig. 2f ) whereas that of USP is in the antagonist position (presence of a phospholipid ligand; Fig. 2e ; ref. 13 ). Regarding the DBD/DNA region, EcR carries a short C-terminal extension (CTE) helix (shorter than in VDR or TR; see comparison in ref. 11 ) which forms at the end of the DBD [14] with natural, functionally relevant EcREs (as used in the present study), whereas it is not visible when an idealized, fully symmetric consensus IR1 is used [16] . The EcR CTE helix is resolved in the map as a prominent feature next to the minor groove of the 3′ half-site ( Fig. 2d ). The CTE identification directly assigns the DNA polarity of the complex, because EcR is known to preferentially bind to the 3′ half-site, whereas USP binds to the 5′ half-site of EcREs [14] , [16] , [17] , [18] , [19] , as confirmed independently by the cryo-EM analysis of an USP/EcR complex with a long 3′-extended DNA RE ( hsp27-3 ′; Figs 1c and 2b ). From the isolated DBD/DNA crystal structure, it is known that the DBDs sit like a saddle on either side of the DNA, rotated around the DNA axis by about 90° when bound to an IR1. The full NR complex reveals here that the LBDs are not ‘sitting’ on the USP DBD because the DBDs are positioned side-on to the DNA ( Fig. 2a ), with the LBDs rotated about 90° clockwise with respect to the DBD ‘saddle’ on the DNA (when viewed from the 3′ side). The 5′-USP DBD thereby connects directly to the LBD (the distance of ~20 Å can be covered by the 19-residue long hinge region), whereas the short CTE of the 3′-EcR ends up on the top of the DNA ( Fig. 2a,c,d ), thus facing the LBDs and facilitating the connection with helix H1 of the EcR LBD. Because of the asymmetric binding of the complex to the DNA, the EcR LBD and DBD are positioned rather far from each other (55 Å) on either 5′- and 3′-ends of the RE, consistent with the 62 residues long linker region of EcR that connects the CTE region with helix H1 at the N-terminal end of the LBD. The precise path of the USP and EcR hinges cannot be resolved in the map, but it appears likely that both are in close vicinity to the DNA. The fact that the hinges provide two independent anchor points on the DNA-bound ‘DBD saddle’ contributes to the stabilization of the complex in a well-defined conformation with respect to the DNA. This observation emphasizes the functionally essential role played by the hinge region and in particular by the CTE in the ligand- and DNA-dependent inter-domain cross-talk. This high level of allostery is consistent with biochemical data showing that the deletion of the EcR CTE fragment encompassing the A-box sequence severely decreases the binding of EcR DBD to hsp27 [18] ; similarly, the CTE and hinge region of homodimeric steroid NRs [20] , monomeric orphan NRs [21] and some heterodimeric NRs bound to direct repeats (VDR, TR) have an important role in transcriptional activation [22] , [23] . Proximity of the USP LBD with the 5′ DNA region An exciting feature of the structure of the USP/EcR DNA complex is the unexpected finding that the USP LBD is in close proximity to DNA because the LBD heterodimer is tilted in the 5′ direction ( Fig. 2a ). To address this in more detail, we determined the structure of the USP/EcR complex with hsp27 extended by five base pairs on the DNA 5′-end ( 5 ′ -hsp27 ; Figs 1b and 3a ). The structure suggests that residues Arg360, Lys394, Arg404 and Arg405 in helix H9 of USP are in contacting distance with the 5′-flanking sequence of the RE. If considering that the DNA would extend further on the 5′ side, it would have to be slightly bent to avoid steric clashes with the USP LBD ( Fig. 3a ). The residues are all surface-exposed residues located in helix H9, which is the part in the LBD furthest away from the ligand-binding pocket and therefore very unlikely to influence ligand affinity. However, because the residues are positively charged, they may be interacting with the negatively charged phosphate backbone of the DNA in a non base-pair-specific manner. We therefore set out to test the functional relevance of these interactions with the 5′ flanking region. We performed transient transfection assays in mammalian HEK293 cells ( Fig. 3b ) that were co-transfected with EcR and wild-type or mutant USP carrying single or multiple alanine substitutions of residues Arg360, Lys394, Arg404 and Arg405 in a luciferase reporter assay. On ponasterone A treatment, a 3- to 4-fold transcriptional activation is seen for wild-type USP, whereas mutating one or several of the residues gradually increases the transcriptional activation fold up to 30–40% ( Fig. 3b ). A similar trend is observed when using the COS-1 cell line ( Supplementary Fig. 6 ). This suggests that these residues are involved in functional interactions that help fine-tuning the transcriptional activity by limiting the inducibility of the ecdysone receptor on ecdysteroid binding. A decrease of the number of interactions would be expected to decrease transactivation; however, the mutations may actually result in de-repression because USP acts as a repressor which involves interactions with the DNA [24] . The gradual increase would be consistent with nonspecific interactions such as those with the DNA phosphate moieties. 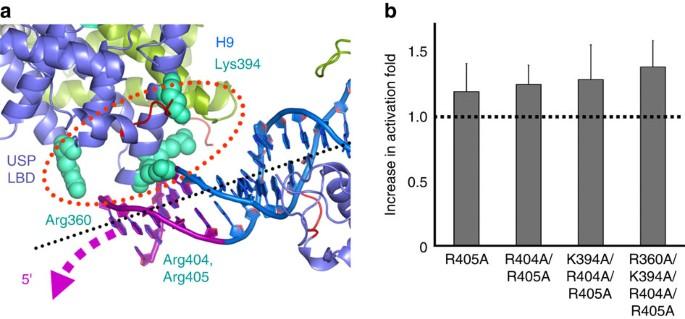Figure 3: Structural and functional analysis of the interactions of USP LBD with the 5′ DNA region. (a) The structure of the USP/EcR/5'-hsp27complex extended by five nucleotides (indicated in magenta) as compared with the USP/EcR/hsp27core complex, revealing that residues Arg360, Lys394, Arg404 and Arg405 (indicated in cyan) in helix H9 of USP LBD are in close proximity of the 5′-flanking region of the RE. USP and EcR LBDs are shown in blue and green, respectively. The arrow indicates the deviation from a linear DNA (dotted line) which would otherwise clash with the USP LBD. (b) Differential effects of alanine-mutations of residues in helix H9 of USP LBD in HEK293 EBNA cells, revealing a gradual increase of the transactivation fold of the single (R405A), double (R404, R405A), triple (K394A, R404, R405A) and quadruple (R360A, K394A, R404, R405A) USP mutants as compared with wild-type USP; see also similar results obtained with COS cells (Supplementary Fig. 6). Error bars refer to the normalized standard deviations in the increase of activation fold for multiple experiments performed in triplicate as described in the Methods part. Figure 3: Structural and functional analysis of the interactions of USP LBD with the 5′ DNA region. ( a ) The structure of the USP/EcR/ 5'-hsp27 complex extended by five nucleotides (indicated in magenta) as compared with the USP/EcR/ hsp27 core complex, revealing that residues Arg360, Lys394, Arg404 and Arg405 (indicated in cyan) in helix H9 of USP LBD are in close proximity of the 5′-flanking region of the RE. USP and EcR LBDs are shown in blue and green, respectively. The arrow indicates the deviation from a linear DNA (dotted line) which would otherwise clash with the USP LBD. ( b ) Differential effects of alanine-mutations of residues in helix H9 of USP LBD in HEK293 EBNA cells, revealing a gradual increase of the transactivation fold of the single (R405A), double (R404, R405A), triple (K394A, R404, R405A) and quadruple (R360A, K394A, R404, R405A) USP mutants as compared with wild-type USP; see also similar results obtained with COS cells ( Supplementary Fig. 6 ). Error bars refer to the normalized standard deviations in the increase of activation fold for multiple experiments performed in triplicate as described in the Methods part. Full size image A general feature of the DNA-bound USP/EcR complex is its open conformation, suggesting that beyond the classical LBD–LBD, DBD–DBD and DBD–DNA interfaces, no additional surfaces are formed in the context of the full complex. The comparison of the IR1-bound USP/EcR complex with that of the DR-bound NRs such as RXR/VDR [11] or HNF4 [10] reveals that the LBDs are also off-centred towards the 5′-end of the RE ( Fig. 4a,b ). This indicates that DR and even essentially symmetric IR REs generate a polarity of the DNA and thus impose an asymmetry to the overall DNA-bound NR complex. This asymmetry appears to be an important feature conserved in the two NR subfamilies, regardless of whether the RE is of DR or steroid-like IR type. However, an important observation here is that the LBD positioning within the LBD heterodimer is inverted in the IR as compared with a DR complex ( Fig. 4b ). This appears to be a direct consequence of the inversion of the second half-site which imposes an inversion of the DBD, a geometrical constraint that is transmitted to the LBD region. Thus, although the open architecture of the USP/EcR/ hsp27 complex is important for the accessibility of co-regulators, the orientation of the coregulator binding-site becomes inverted as well. The LBD inversion is functionally highly relevant, because the co-regulator preferentially bind to the partner of RXR (or USP), for example, the insect-specific TAIMAN coactivator binds to EcR [25] , and DRIP/SRCs binds the VDR part of RXR/VDR heterodimers [9] . As a consequence, the co-regulator binding-site will face opposite orientations in IR- and DR-bound NR complexes, suggesting that the DNA topology is a major driver in the formation of specific coregulator complexes (summarized schematically in Fig. 4c ). The 3D visualization thus provides new concepts that can be probed in future experiments, such as the possible influence of asymmetry on the activity of co-activators. 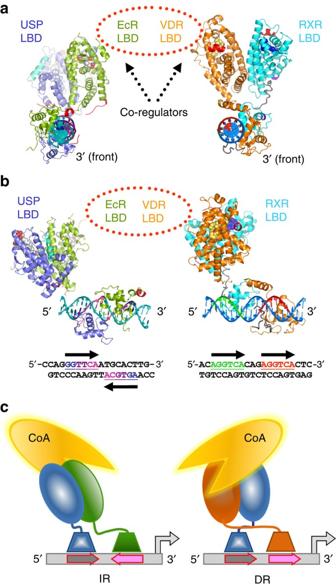Figure 4: Topology of IR- and DR-bound nuclear receptor complexes. (a,b) 3′-end and side-views of the USP/EcR/hsp27complex bound to an IR1 RE as compared with the RXR/VDR complex bound to a DR3 RE11. The inversion of the second half-site sequence between DR and IR REs imposes a flip of the LBDs, leading to an inversion of the orientation of the binding site for the recruitment of chromatin-modifying co-regulator proteins. (c) Schematic representation of the LBD inversion that is observed between the IR- and DR-bound USP/EcR and RXR/VDR complexes, illustrating a strong DNA-dependent allostery that defines the orientation of co-regulators (shown in orange and labelled CoA). Figure 4: Topology of IR- and DR-bound nuclear receptor complexes. ( a , b ) 3′-end and side-views of the USP/EcR/ hsp27 complex bound to an IR1 RE as compared with the RXR/VDR complex bound to a DR3 RE [11] . The inversion of the second half-site sequence between DR and IR REs imposes a flip of the LBDs, leading to an inversion of the orientation of the binding site for the recruitment of chromatin-modifying co-regulator proteins. ( c ) Schematic representation of the LBD inversion that is observed between the IR- and DR-bound USP/EcR and RXR/VDR complexes, illustrating a strong DNA-dependent allostery that defines the orientation of co-regulators (shown in orange and labelled CoA). Full size image Taken together, by elucidating the architecture of three USP/EcR DNA complexes ( Fig. 1 ), this study provides insights into the structural determinants of heterodimeric and steroid-like NRs bound to IR DNA elements. It reveals that the IR-bound complex adopts a highly asymmetric organization which stands in contrast to the symmetric nature of the DNA. Thus, the concept that emerges from our study is that, regardless of polar DR or (pseudo-)symmetric IR REs, the NR dimer adopts an asymmetric organization with respect to the two half-sites of the RE ( Fig. 4 ). The observed LBD domain flip between the DR and IR complexes and the asymmetry of the palindromic DNA complex thus seem to be imprinted in the sequence of the DNA RE, a mechanism which is reminiscent of a DNA-dependent allostery that in fine defines the overall topology and the specific position of the coregulator-binding NR subunit of the complex. Finally, through a structural and functional analysis of several USP/EcR/DNA complexes, we show that the USP LBD region unexpectedly contributes to a 5′-extended DNA-binding-site located next to the core RE, which, together with the DBDs, helps to stabilize the complex on the DNA and fine-tune gene regulation. A key, unexpected finding of our study is that a dimeric protein complex adopts an asymmetric organization even though it is bound to a symmetric DNA. That this applies in general for homo- and heterodimer and is not due to the mere presence of a heterodimer is illustrated by the fact that the DNA induces an LBD flip in the heterodimeric USP/EcR and RXR/VDR complexes when the orientation of the second half-site is reversed (IR versus DR; Fig. 4b ). This concept is of interest for protein–DNA complexes in general and of striking importance for understanding NR function in particular. Indeed, no full-length NRs have been studied when bound to a palindromic DNA. The current textbook understanding is that such complexes would be symmetric (this is the way they are usually drawn in schemes). However, the asymmetric organisation revealed here ( Fig. 4 ) has important functional consequences. Indeed, symmetric and near-symmetric DNA segments represent the type of REs bound by NRs of the steroid family. Thus, deciphering the function of DNA with respect to transcription regulation is important in the context of the recognition by steroid NRs of co-regulator proteins (co-repressors and co-activators). In fact, as a consequence of the asymmetry of the NR–DNA complex, co-regulators are oriented in a particular way for chromatin remodelling. This study therefore provides the first direct evidence of the role of the DNA—palindromic as opposed to DRs studied in the past—on the architecture of full NRs. These novel insights on palindrome-bound complexes were made possible because of the analysis of a full NR complex as opposed to studies limited to sole DBD–DNA complexes. In fact, focusing on the palindrome-bound DBD structures might give a misleading impression of symmetry that does not apply to the entire complex. Finally, an advantageous aspect related to the study of a dimeric receptor comprising two different proteins (USP and EcR) is that the asymmetry of the protein complex bound to a symmetric DNA can be addressed in an unambiguous manner, because the two subunits can be distinguished within the complex. In contrast, for a homodimeric NR complex with two identical proteins, such as ER/ER, this would prove to be difficult because of the ambiguity in terms of the connectivity between LBD and DBD of each monomer (the hinge region is often undefined in previous structures because of its flexible character). Thus, the USP/EcR complex is a valuable model system to analyse NR-bound inverted repeats. Furthermore, its structure represents a major conceptual advance in the field by suggesting that not only hetero-, but also homodimeric NRs are likely to adopt an asymmetric conformation and behave as heterodimers when bound to DNA, thus illustrating the role of DNA in allosterically positioning the LBDs. Cloning, protein expression and purification H. virescens HvEcR-B ΔAB (139–532) was cloned into a pET-derived expression vector, containing an N-terminal hexahistidine tag, and H. virescens HvUSP ΔAB (103–466) was cloned into a pACYC11b plasmid encoding a native protein (the AB domains were removed because of their highly variable and unstructured character). The two constructs were co-expressed in Escherichia coli BL21 (DE3) strains. Cells growing in sucrose-enriched media were induced at 18 °C overnight with 1 mM of IPTG in the presence of 1 mM of the ecdysteroid analogue BYI06830 from Bayer CropScience (Leverkusen, Germany) dissolved in dimethylsulphoxide [13] . The cells were harvested, sonicated and centrifuged in a buffer containing 20 mM TRIS/HCl pH=8.0, 250 mM KCl, 250 mM NaCl, 4 mM CHAPS, 10% glycerol, 5 mM imidazole. The supernatant was loaded on 5 ml HisTrap FF crude column (GE Healthcare). The proteins were eluted at 250 mM imidazole and further purified by size-exclusion chromatography on Superdex S200 (16/60 and 10/300, GE Healthcare) columns. The final buffer was 10 mM TRIS pH 7.5, 100 mM NaCl, 10 mM MgCl 2 , 10 mM TCEP. Protein samples were concentrated using Amicon-Ultra centrifugal filter units (Millipore). Complexes of USP/EcR and REs were formed by adding a 1.3-fold molar excess of DNA to the receptor heterodimer followed by an additional gel filtration step. Purity and homogeneity of the proteins were assessed by SDS–polyacrylamide gel electrophoresis and complex formation was monitored by native polyacrylamide gel electrophoresis. The DNA oligonucleotides used for our experiments are derived from the promoter of the hsp27 gene and have the following sequences: (i) hsp27 : 5′-CCAG GGTTCA A TGCACT TG-3′ for the forward strand and 5′-CCAAGTGCATTGAACCCTG-3′ for the reverse strand, (ii) hsp27-3 ′: 5′-AG GGTTCA A TGCACT CT CGCATATATTAGGCGGCG -3 ′ for the forward strand and 5′- CGCCGCCTAATATATGCG AGAGTGCATTGAACCCT-3′ for the reverse strand, (iii) 5'-hsp27 : 5 ′- CGAGA CAAG GGTTCA A TGCACT TG-3′ for the forward strand and 5′-CAAGTGCATTGAACCCTTG TCTCG -3′ for the reverse strand (RE half-sites are underlined and 5′- and 3′-extensions are italicized). Cryo electron microscopy Sample freezing and image processing follow the procedures described in refs 11 , 26 . In brief, samples of the USP/EcR/ hsp27 complex were plunge-frozen on holey carbon QUANTIFOIL EM grids using a Vitrobot Mark IV (FEI) to embed the complex in a thin film of vitrified buffer spanning the holes of the carbon film after blotting the excess solution and freezing the grids into liquid ethane. Images were collected at liquid nitrogen temperature with the in-house FEI Polara FEG cryo electron microscope at 100 kV acceleration voltage with a dose of 20 electrons/Å 2 at a magnification of 59,000 on a 4 k × 4 k CCD camera (FEI Eagle) with a pixel size of 1.96 Å. Focal-pair images −1.5 to −3 μm versus −5 to −7 μm underfocus were collected. CTF correction was done using the Imagic-V software package [27] , [28] . Particle selection from the far-from-focus images with individual validation by visual inspection was performed with the boxer routine of the EMAN software package [29] . A total of 4,936 single particles from the far-from-focus images were used for an ab initio 3D reconstruction (see ref. 11 ) by angular reconstitution using the cross common line approach applied to class average images and validated by comparison of the re-projections with the original particle images and class averages. The obtained structure was refined iteratively with only close-to-focus data (50,000 particles selected from 600 CCD images) using the cross common lines approach as described previously [11] , [26] . The resolution of the final USP/EcR/ hsp27 3D reconstruction was estimated with the Fourier Shell Correlation [30] according to the 0.5, one-half-bit [31] and 0.143 (ref. 32 ) criteria to 11.6/9.2/8.7 Å consistent with the features of the map. Data for the USP/EcR/ 5'-hsp27 complex were collected and processed in the same way using 10,786 particles from 97 CCD images; the structure was determined ab initio using the C1 startup procedure of Imagic-V, independently of the USP/EcR/ hsp27 complex. For the USP/EcR/ hsp27-3 ′ complex, the sample (0.5 mg ml −1 ) was flash-frozen using a home-made plunge-freezer and 120 photographic films (Kodak SO-163) were recorded using the in-house transmission electron microscope (FEI Tecnai F20) operating at 200 kV. Micrographs were digitized with a high-precision drum scanner (Heidelberger Druckmaschinen) resulting in a final step size of 1.0 Å per pixel (scanning step size 4.66 μm). After particle selection (31,000) and CTF correction, the images were coarsened three times resulting in spatial a resolution of 3.0 Å per pixel for further image processing. The structure was refined using the Imagic-V software with the structure of the USP/EcR hsp27 complex as an initial reference. After a few refinement cycles, the additional density corresponding to the 3′-extended DNA was clearly visible. Map interpretation The interpretation of the 3D density map was done by fitting the individual crystal structures of the USP/EcR LBD and DBD heterodimers, respectively (PDB IDs 1R1K and 2HAN; [13] , [14] ) taking into account the connectivity between the two major parts of the complex. Final pixel sizes after magnification calibration with the fitted crystal structures is 1.8 Å for the USP/EcR/ hsp27 and USP/EcR/ hsp27-5 ′ complexes, and 2.8 Å for the USP/EcR/ hsp27-3 ′ complex. Fitting and preparation of figures was done using the PyMOL software ( http://pymol.sourceforge.net ). The cryo-EM map and the fitted coordinates were deposited in the EM and protein data bank under accession numbers EMD-2631 and PDB ID 4UMM . Small-angle X-ray scattering Synchrotron X-ray solution scattering data were collected at the SWING beamline at SOLEIL Synchrotron (Gif-sur-Yvette, France), using an HPLC-coupled SAXS cell and a 17 × 17 cm 2 low-noise Aviex CCD detector positioned at a distance of 2.107 m from the sample. Sample solutions were circulated in a thermostated Quartz capillary with a diameter of 1.5 mm and 10 μm wall thickness, positioned within a vacuum chamber. About 20–40 μl protein were injected at relatively high concentrations (4–10 mg ml −1 ) into a size-exclusion chromatography column (SHODEX KW402.5), using an Agilent HPLC system and eluted directly into the SAXS flow-through capillary cell at a flow rate of 200 μl min −1 (ref. 33 ). SAXS data were collected online throughout the whole elution time, with 1.5 s frame duration and 0.5 s dead time between frames. In total, 250 frames were collected and normalized to transmitted intensity. The frames corresponding to the elution peak of the complex were averaged using ‘Foxtrot’, a dedicated home-made application. The SAXS data were processed using standard procedures in the program package PRIMUS [34] . The forward scattering I (0) and the radii of gyration Rg were evaluated using the Guinier approximation, assuming that at very small angles Q <1.3/Rg, the intensity is represented as I ( Q )= I (0) exp(−(1/3)( Q Rg) 2 ). The maximum dimensions Dmax were computed using the indirect transform package GNOM [35] which provides the distance distribution functions p ( r ). Low resolution shape analysis of the solutes was performed using the ab initio program DAMMIF [36] which represents the macromolecule by an assembly of densely packed beads and employs simulated annealing to build a compact interconnected configuration of beads that fits the experimental data I exp( Q ). The scattering from the atomic models was calculated using the program CRYSOL 2.7 (ref. 37 ; without constant subtraction), which either predicts theoretical scattering patterns using a default hydration layer density or fits the experimental data by adjusting the excluded volume and the contrast of the hydration layer. The discrepancy factor χ 2 between experimental intensities and calculated intensities from the models at each value of momentum transfer Q was calculated as follows: χ 2 =1/( n −1)∑ j [( I exp( Qj )− k ′ I calc( Qj ))/ σ ( Qj )] 2 , where n is the number of experimental points, k a scaling factor, and I exp( Qj ) the experimental intensity, I calc( Qj ) the calculated intensity and σ ( Qj ) the experimental error. The corresponding reduced residuals of the fit are the individual terms in the above equation and assess the quality of the fit over the whole Q range. Cell cultures Human embryonic kidney 293 EBNA cells were cultured in Dulbecco’s modified Eagle’s medium. The medium was supplemented with 10% heat-inactivated fetal calf serum, gentamycin and G418 sulphate at 37 °C under 5% CO 2 humidified atmosphere. African Green Monkey Cercopithecus aethiops fibroblast-like kidney (COS-1) cells were cultured in Dulbecco’s modified Eagle’s medium. The medium was supplemented with 5% heat-inactivated fetal calf serum and gentamycin at 37 °C under 5% CO 2 humidified atmosphere. Transfection assays Transient transfection assays were carried out in 24-well plates (10 5 cells per well) using the standard jetPEI (Polyplus-transfection, Illkirch, France) transfection protocol. HEK293 EBNA (or alternatively COS-1) cells were co-transfected with 100 ng full-length HvEcR-B (1-558) and 100 ng HvUSP (1-466) pCMX expression plasmids, 100 ng pGL3-minTK-hsp27(3x)-fireflyLUC reporter vector and 2 ng pRLTR Renilla LUC expression plasmid. The pCMX expression plasmids were provided by Bayer CropScience (Leverkusen, Germany). The pGL3-minTK-hsp27(3x)-fireflyLUC vector is a modified version of the pGL3-Basic luciferase reporter vector (Promega Corporation) and comprises a minimal thymidine kinase minimal promoter inserted before the luciferase gene using the HindIII and NcoI restriction sites and three copies of a 48 bp long fragment of the hsp27 gene promoter encompassing the IR1 EcRE. For the insertion of the hsp27 EcRE element in the pGL3minTK plasmid, the plasmid was digested by NheI and XhoI and a primer hybrid (hsp27 × 1-F/hsp27 × 1-R) was inserted. For the insertion of an extra copy of the hsp27 EcRE, pGL3minTK-hsp27v1 (one copy) and pGL3minTK-hsp27v2 (two copies) were digested by NheI and a primer hybrid (hsp27 × 1-F/hsp27 × 1-R) was inserted. Primer sequences: forward, hsp27 × 1-F: 5′-CTAGGcgaagcgagacaagggttcaatgcacttgtccGCTAGCTAGC–3′; reverse, hsp27 × 1-R: 5-TCGAGCTAGCTAGCGGACAAGTGCATTGAACCCTTGTCTCGCTTCGC-3′. Cells were treated with 5 × 10 −6 M ponA for 18 h and cell extracts were assayed for firefly and Renilla luciferase activities using the Dual-LuciferaseR Reporter Assay (Promega Corporation), as described in the manufacturer’s protocol. Firefly luciferase values were normalized to Renilla luciferase activity. Data points represent the mean of assays performed as four independent experiments for the quadruple mutant, three for the double and the triple and two for single mutants, each being performed in triplicate ( Fig. 3b ). The error bars refer to the normalized standard deviations ( , where N is the number of experiments) in the increase of activation fold for multiple experiments performed in triplicate as described in the Methods part. Mutants were generated using the QuickChange site-directed mutagenesis kit from Stratagene. Primer sequences for mutant design: R360A forward: AAGATGCGCACCCTGGCCGTCGACCAGGCCGAG; reverse: CTCGGCCTGGTCGACGGCCAGGGTGCGCATCTT; K394A: forward: GAAGTTTTACGAGAAGCGATGTTCCTGTGCCTG; reverse: CAGGCACAGGAACATCGCTTCTCGTAAAACTTC; R404A: forward: CTGGACGAGTACTGCGCCCGCTCGCGCAGTTCG; reverse: CGAACTGCGCGAGCGGGCGCAGTACTCGTCCAG; R405A: forward: GACGAGTACTGCCGCGCCTCGCGCAGTTCGGAG; reverse: CTCCGAACTGCGCGAGGCGCGGCAGTACTCGTC; R404A/R405A: forward: CTGGACGAGTACTGCGCCGCCTCGCGCAGTTCGGAG; reverse: CTCCGAACTGCGCGAGGCGGCGCAGTACTCGTCCAG. All mutants were confirmed by sequence analysis. Transfection assays with COS-1 cells were performed as for HEK293 EBNA cells and show the same trend as for the HEK293 assays ( Supplementary Fig. 6 ). How to cite this article: Maletta, M. et al . The palindromic DNA-bound USP/EcR nuclear receptor adopts an asymmetric organization with allosteric domain positioning. Nat. Commun. 5:4139 doi: 10.1038/ncomms5139 (2014). Accession codes: The electron density map and the fitted coordinates of the USP/EcR DNA complex have been deposited in the EM Data Bank under the accession number EMD-2631 and in the Protein Data Bank under the accession number 4UMM .